Tailoring the hydrophobicity of graphene for its use as nanopores for DNA translocation Graphene nanopores are potential successors to biological and silicon-based nanopores. For sensing applications, it is however crucial to understand and block the strong nonspecific hydrophobic interactions between DNA and graphene. Here we demonstrate a novel scheme to prevent DNA–graphene interactions, based on a tailored self-assembled monolayer. For bare graphene, we encounter a paradox: whereas contaminated graphene nanopores facilitated DNA translocation well, clean crystalline graphene pores very quickly exhibit clogging of the pore. We attribute this to strong interactions between DNA nucleotides and graphene, yielding sticking and irreversible pore closure. We develop a general strategy to noncovalently tailor the hydrophobic surface of graphene by designing a dedicated self-assembled monolayer of pyrene ethylene glycol, which renders the surface hydrophilic. We demonstrate that this prevents DNA to adsorb on graphene and show that single-stranded DNA can now be detected in graphene nanopores with excellent nanopore durability and reproducibility. The idea of nanopore-based DNA analysis and sequencing is that a nanopore, a tiny hole in a membrane, can be used as a nanoscale recorder that scans a single DNA molecule from head to tail to ultimately read off the genetic information—for example, using the ion current passing through the pore to probe the identity of the base. In the last decade, many groups have developed strategies to detect DNA molecules using nanopores to understand the biophysics of DNA translocation [1] , [2] , [3] . Only very recently, it was demonstrated that biological nanopores can be used to obtain sequence information if a DNA polymerase is used to slowly ratchet the DNA through the pore [4] , [5] . Graphene nanopores were introduced in 2010 (refs 6 , 7 , 8 ). Graphene forms the ultimate nanopore membrane, as it is a hexagonal carbon sheet with a thickness of only a single atom, and yet it is fully preventing ion transport across the monolayer membrane. Furthermore, it is electrically conductive, which opens up new modalities of directly probing the chemical nature of the bases—for example, by running a tunnelling current through the DNA molecule that is traversing a graphene gap [9] , [10] , [11] . To pursue such an approach, it is crucial to maintain the crystallinity of graphene right up to the edges of the nanopore. Indeed, future graphene devices—those, for instance, involving nanogaps or ribbons were theoretically predicted to have DNA-sequencing capabilities if graphene remains unaltered electrically by conserving its crystallinity [10] , [12] . In this paper, we report that DNA translocation of single-stranded and double-stranded DNA is difficult when graphene nanopores are clean and crystalline because of severe clogging and sticking of DNA. We therefore develop a general approach to modify the hydrophobicity of graphene with non-covalently bound hydrophilic functional groups. We aim for non-covalent rather than covalent functionalization, as the latter would lead to strong changes of the graphene electronic structure that would alter the beneficial conductive properties, as it was noticed earlier for carbon nanotubes [13] , [14] . Crystalline graphene nanopores by in situ heating In the first publications on graphene nanopores, pores were fabricated at room temperature by locally bombarding a graphene monolayer with a focused 300-keV electron beam [6] , [7] , [8] . As shown in Fig. 1a , these conditions yield the deterioration of the graphene lattice with increasing beam exposure time (as evidenced by the loss of the characteristic hexagonal diffraction pattern of graphene; Fig. 1a , situations 1–3). By exposing graphene at temperatures above 500 °C in the STEM (scanning transmission electron microscopy) mode of a TEM (transmission electron microscopy) [15] , [16] , however, it has recently become possible to preserve the graphene lattice up to the edges of the nanopore ( Fig. 1b ). This result is similar to what has been achieved by Zettl et al . [17] , although our process allows good control over the size and shape of the nanostructure being patterned. 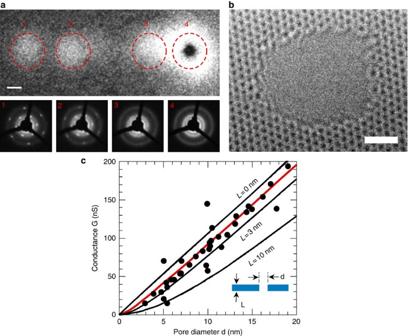Figure 1: Crystallinity and ionic conductance of graphene nanopores. (a) Amorphization and contamination of a graphene monolayer induced by a focused electron beam at room temperature during nanopore drilling. Nanopore drilling was carried using an FEI Titan TEM, equipped with Csimage corrector, at 300 kV, spot size 4 and C2 aperture 20 μm, on the same graphene layer. The electron beam, focused into a 10-nm sized probe, was exposed on graphene with increased residence time of 10, 20, 30 and 40 s for situations 1–4, respectively. After the intermediate stages 1–3, a pore was formed at stage 4. After the electron-beam exposure, nano-electron diffraction patterns were taken (see bottom panel (scale bar is 10 nm)). (b) HREM image (80 kV) of a 3-nm nanopore with clean and crystalline edge drilled in STEM mode at 600 °C using an FEI Titan 60–300 PICO TEM equipped with a high brightness electron gun, an electron gun monochromator, a probe aberration corrector and a CS-CCachro-aplanat image corrector (scale bar is 1 nm). (c) Dependence of the conductance of crystalline nanopores on pore diameter. Black lines represent a model of conductance (Equation 1) forL=0, 3 and 10 nm, whereLrepresents the thickness of the nanopore membrane. The solid red line represents the best fit (lowest reducedχ2) forL=1.2±0.1 nm. Figure 1: Crystallinity and ionic conductance of graphene nanopores. ( a ) Amorphization and contamination of a graphene monolayer induced by a focused electron beam at room temperature during nanopore drilling. Nanopore drilling was carried using an FEI Titan TEM, equipped with C s image corrector, at 300 kV, spot size 4 and C2 aperture 20 μm, on the same graphene layer. The electron beam, focused into a 10-nm sized probe, was exposed on graphene with increased residence time of 10, 20, 30 and 40 s for situations 1–4, respectively. After the intermediate stages 1–3, a pore was formed at stage 4. After the electron-beam exposure, nano-electron diffraction patterns were taken (see bottom panel (scale bar is 10 nm)). ( b ) HREM image (80 kV) of a 3-nm nanopore with clean and crystalline edge drilled in STEM mode at 600 °C using an FEI Titan 60–300 PICO TEM equipped with a high brightness electron gun, an electron gun monochromator, a probe aberration corrector and a C S -C C achro-aplanat image corrector (scale bar is 1 nm). ( c ) Dependence of the conductance of crystalline nanopores on pore diameter. Black lines represent a model of conductance (Equation 1) for L =0, 3 and 10 nm, where L represents the thickness of the nanopore membrane. The solid red line represents the best fit (lowest reduced χ 2 ) for L =1.2±0.1 nm. Full size image We fabricated graphene nanopores using this approach, with diameters from 3 to 20 nm. The diameter of the nanopore was determined as the square root of the measured area of the nanopore (see Supplementary Fig. S1 for an overview of some representative nanopores). Subsequently, we probed the ionic conductance of these pores in a buffer containing 1 M KCl and 10 mM Tris (pH 8.1). Figure 1c plots the conductance values of these nanopores versus the pore diameter. As expected, the conductance of the nanopore increases for increasing pore diameter. A simple model [18] describes the conductance G of the pore with diameter d in a buffer of conductivity σ as the inverse sum of the access resistance contribution and the resistance of a cylinder with length L , A fit of Equation 1 shows that the conductance values are distributed between L =0 nm and L =3 nm, with a best fit (lowest reduced χ 2 ) at L =1.2±0.1 nm. This contrasts the earlier data, where G ( d ) was best fitted by much larger value of L =9 nm (ref. 6 ) and indicates that indeed the new high-temperature STEM method results in much cleaner graphene. Crystalline graphene nanopores clogged with DNA Surprisingly, if these crystalline nanopores ( Fig. 1c ) are used to detect DNA molecules, severe clogging is experienced, as observed by a stepwise decrease in ionic current of the nanopore and subsequent irreversible pore closure. As seen in Fig. 2a , a few translocation events were observed for a couple of seconds after addition of the DNA. Then, however, the open pore current dropped to zero, signifying a closed, irreversibly clogged pore. Even 1-V pulses were not sufficient to unclog the pore. We imaged this particular pore before and after clogging (see Fig. 2b,c , respectively). After use, DNA material is clearly visible on the STEM micrographs as a white blob-like aggregate in the pore, along with the fibril-like structures around the pore. 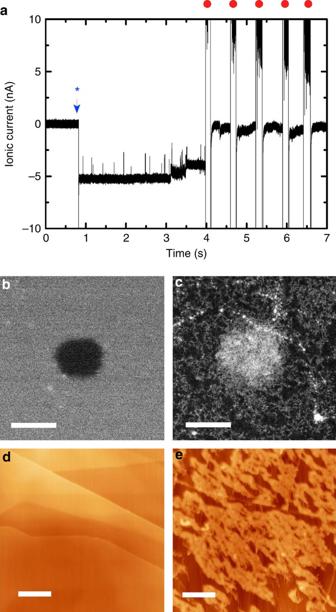Figure 2: DNA molecules clog crystalline graphene nanopores. (a) Ionic current versus time of a 5-nm diameter graphene nanopore incubated with single-stranded DNA M13 at a concentration of 2.5 ng μl−1in 1 M KCl and 8 M urea. At time 0.7 s (blue star), the voltage is switched from 0 to −200 mV, resulting in a baseline current of −5.2 nA and upward peaks corresponding to DNA translocation events. After 2 s at −200 mV, the current baseline starts to decrease towards zero in discrete steps, quickly leading to a full clogging of the pore. Large 1 V pulses (red dots) are subsequently applied across the nanopore in order to try to restore the stable current baseline; however, this was unsuccessful. (b) The 5-nm nanopore discussed in panel A before the translocation of DNA (scale bar is 5 nm) and (c) the same nanopore after the experiment that showed pore clogging, both imaged in the STEM mode of the TEM (scale bar is 5 nm). (d) AFM of highly oriented pyrolitic graphite (HOPG) incubated for 5 min with a solution of 3 M KCl and 8 M urea and rinsed with ultrapure water (scale bar is 200 nm). (e) HOPG incubated for 5 min with single-stranded M13 DNA (10 ng μl−1) in the same buffer (scale bar is 200 nm). Symbol * corresponds to the time at which the voltage is applied (i.e., when the baseline current shilfs). Figure 2: DNA molecules clog crystalline graphene nanopores. ( a ) Ionic current versus time of a 5-nm diameter graphene nanopore incubated with single-stranded DNA M13 at a concentration of 2.5 ng μl −1 in 1 M KCl and 8 M urea. At time 0.7 s (blue star), the voltage is switched from 0 to −200 mV, resulting in a baseline current of −5.2 nA and upward peaks corresponding to DNA translocation events. After 2 s at −200 mV, the current baseline starts to decrease towards zero in discrete steps, quickly leading to a full clogging of the pore. Large 1 V pulses (red dots) are subsequently applied across the nanopore in order to try to restore the stable current baseline; however, this was unsuccessful. ( b ) The 5-nm nanopore discussed in panel A before the translocation of DNA (scale bar is 5 nm) and ( c ) the same nanopore after the experiment that showed pore clogging, both imaged in the STEM mode of the TEM (scale bar is 5 nm). ( d ) AFM of highly oriented pyrolitic graphite (HOPG) incubated for 5 min with a solution of 3 M KCl and 8 M urea and rinsed with ultrapure water (scale bar is 200 nm). ( e ) HOPG incubated for 5 min with single-stranded M13 DNA (10 ng μl −1 ) in the same buffer (scale bar is 200 nm). Symbol * corresponds to the time at which the voltage is applied (i.e., when the baseline current shilfs). Full size image We hypothesize that the clogging is because of DNA that sticks to the graphene. To investigate this, we studied single-stranded DNA on graphite with atomic force microscopy (AFM). When DNA is incubated in solution on the surface of graphite ( Fig. 2d ), it indeed adsorbs strongly on the surface, as seen by the appearance of 1.2±0.2 nm high patches on AFM images ( Fig. 2e ). It is long known that DNA adsorbs well on graphite [19] , [20] , [21] , [22] . Presumably, the aromatic purine and pyrimidine bases in DNA molecules drive the DNA molecules towards irreversible adsorption on the surface of graphene. To counteract such adsorption phenomena, Garaj et al . [8] proposed earlier that a very high salt concentration (buffers containing 3 M KCl) might prevent DNA (single-stranded as well as double-stranded) from adsorbing to graphene. This is however contradicted by our observations with single-stranded DNA ( Fig. 2d at 3 M KCl) and double-stranded DNA (at KCl concentrations of 1 and 3 M, and different pH ranging from 8 to 12). Whereas such DNA–graphene interactions may be desirable in some sensor devices, they must be prevented in nanopore translocation, in which each nucleobase should slide unimpededly through the nanopore as opposed to sticking irreversibly to the graphene surface. Note also that wrinkles are known to form within graphene that is transferred on a flat substrate [23] . Although we do not expect wrinkles to have a role in the adsorption of DNA on graphene, we cannot rigorously exclude this. Self-assembled hydrophilic monolayer coating To address the issue that clean crystalline graphene nanopores get clogged in the presence of DNA, we designed a dedicated self-assembled monolayer. This self-assembled hydrophilic coating aims at preventing DNA to adsorb near the nanopore. Note that, whereas the hydrophilic edges of the nanopore will not drive DNA adsorption, hydrophobic interactions at the graphene surface in the proximity of the nanopore will still yield pore clogging in the absence of a coating. Our self-assembled monolayer is based on the combination of two chemicals, namely, a hydrophobic aminopyrene molecule and a hydrophilic N -hydroxysuccinimide derivative of a 4-mer ethylene glycol molecule (that is, tetraethyleneglycol monomethyl ether N -hydroxysuccinimide ester, see Fig. 3a ). Whereas the pyrene moiety will non-covalently stick to the graphene, the ethylene glycol will stick out into the solution and render the surface hydrophilic. Note that this non-covalent self-assembled passivation scheme keeps the graphene material intact from the chemical and electrical degradations that would result from covalent passivation, and importantly, such non-covalent self-assembly can be expected to not affect the electronic conduction of graphene in a significant way [13] , [14] . The coating is applied in two steps from two successive 10-mg ml −1 solution of both molecules in methanol. In a first step, π-stacking interactions drive the adsorption of a monolayer of aminopyrene on graphene. This is followed by the aminolysis of the N-hydroxysuccinimide ester on the carbonyl group (blue, Fig.. 3aii ) by the primary amine on the pyrene molecule (red, Fig. 3ai ), forming a chemically stable peptide NHCO bond between the two molecules ( Fig. 3a , bottom). We decided for a two-step reaction to provide more efficient π-stacking of the pyrene–NH 2 to the graphene surface in the first step and thus avoid competing adsorption of EG chains. The chemistry for amide formation between NHS and NH 2 is well known from bulk studies. 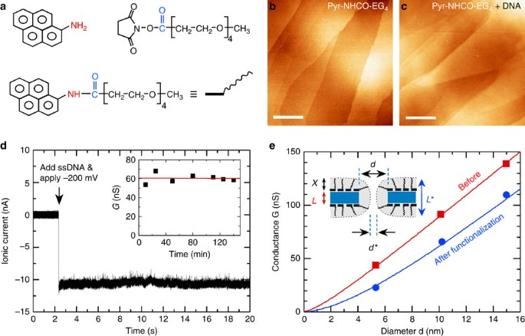Figure 3: Hydrophilic functionalization of the graphene surface provides DNA antifouling. (a) Chemical structures of 1-aminopyrene (top left), a N-hydroxysuccinimide ester derivative of a 4-mer ethylene glycol molecule (top right), and the product of the chemical reaction of both (bottom). (b) HOPG coated with a self-assembled monolayer made of the product of the reaction between 1-aminopyrene and the 4-mer ethylene glycol and incubated with 1 M KCl and 8 M urea in absence of DNA (scale bar is 200 nm). (c) Same as (b) after 10 min of subsequent incubation with the same buffer containing 10 ng μl−1of single-stranded M13 (scale bar is 200 nm). (d) Representative raw time trace of the ionic current versus time for a 14-nm diameter graphene nanopore coated with the self-assembled-monolayer and incubated with single-stranded DNA M13 at a concentration of 10 ng μl−1in 1 M KCl and 8 M urea, showing a clear contrast toFig. 2a. The inset represents the variation in the conductance of the nanopore versus time. (e) Conductance of graphene pores versus diameter before (red squares) and after applying the self-assembled monolayer (blue circles). The red solid line corresponds to a fit of Equation 1, yieldingL=1.5 nm. The blue solid line is a fit of Equation 2, yieldingx=0.7 nm. Conductance measurements were all carried out after DNA incubation. Symbol * corresponds to the time at which the voltage is applied (i.e., when the baseline current shilfs). Figure 3: Hydrophilic functionalization of the graphene surface provides DNA antifouling. ( a ) Chemical structures of 1-aminopyrene (top left), a N-hydroxysuccinimide ester derivative of a 4-mer ethylene glycol molecule (top right), and the product of the chemical reaction of both (bottom). ( b ) HOPG coated with a self-assembled monolayer made of the product of the reaction between 1-aminopyrene and the 4-mer ethylene glycol and incubated with 1 M KCl and 8 M urea in absence of DNA (scale bar is 200 nm). ( c ) Same as ( b ) after 10 min of subsequent incubation with the same buffer containing 10 ng μl −1 of single-stranded M13 (scale bar is 200 nm). ( d ) Representative raw time trace of the ionic current versus time for a 14-nm diameter graphene nanopore coated with the self-assembled-monolayer and incubated with single-stranded DNA M13 at a concentration of 10 ng μl −1 in 1 M KCl and 8 M urea, showing a clear contrast to Fig. 2a . The inset represents the variation in the conductance of the nanopore versus time. ( e ) Conductance of graphene pores versus diameter before (red squares) and after applying the self-assembled monolayer (blue circles). The red solid line corresponds to a fit of Equation 1, yielding L =1.5 nm. The blue solid line is a fit of Equation 2, yielding x =0.7 nm. Conductance measurements were all carried out after DNA incubation. Symbol * corresponds to the time at which the voltage is applied (i.e., when the baseline current shilfs). Full size image We characterized the DNA-passivation properties of the self-assembled monolayer using AFM. Importantly, we found that DNA did not adsorb on graphite that was coated with the self-assembled monolayer, even at concentrations of DNA as high as 10 ng μ −1 . This is evidenced by the similarities between the AFM image before the addition of DNA ( Fig. 3b , self-assembled monolayer on highly oriented pyrolitic graphite incubated with 10 mM Tris, 1 M KCl, 8 M urea, pH 8.1 for 10 min) and after the addition of the same buffer with 10 ng μl −1 of single-stranded DNA ( Fig. 3c ). The self-assembled monolayer thus appears to act as an effective hydrophilic barrier that prevents the hydrophobic interaction between nucleobases in DNA and the aromatic graphene. Most importantly, using this strategy, we were able to reproducibly translocate single-stranded DNA without pore clogging, with experimentation times now measuring in hours rather than seconds, as evidenced by the stable conductance levels versus time ( Fig. 3d and inset). We attribute the stability of the conductance value (with long-term variations of <10%) to a good stability of the coating, which apparently does not get displaced by the presence of the DNA molecules or their translocation under the applied electric field. Importantly, the drastic change in DNA adsorption ( Fig. 2a versus Fig. 4a and Supplementary Fig. S2 ) shows that the coating provides a successful antifouling strategy. As shown in the supporting information ( Supplementary Fig. S2 ), pores of different diameters in the range 5–14 nm behaved in a similar way. 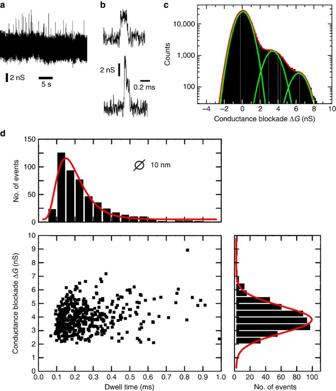Figure 4: DNA translocation through a coated 10-nm graphene nanopore. (a) Translocation of circular M13 single-stranded DNA across a 10-nm nanopore in a graphene monolayer, recorded at full bandwidth. (b) Examples of translocation events of non-folded (type 1, top panel) and partially folded DNA (type 21, bottom panel) molecules recorded at −200 mV in this 10-nm pore. (c) Conductance histogram collected from 545 translocation events, including the open-pore conductance before and after the event. (d) Scatter diagram of the amplitude of the conductance blockade versus translocation time for DNA translocation through a 10-nm diameter nanopore in a graphene monolayer. The accompanying histograms are included at the top and the right. Each point in this scatter diagram corresponds to a single translocation event. Applied voltage is −200 mV. Figure 4: DNA translocation through a coated 10-nm graphene nanopore. ( a ) Translocation of circular M13 single-stranded DNA across a 10-nm nanopore in a graphene monolayer, recorded at full bandwidth. ( b ) Examples of translocation events of non-folded (type 1, top panel) and partially folded DNA (type 21, bottom panel) molecules recorded at −200 mV in this 10-nm pore. ( c ) Conductance histogram collected from 545 translocation events, including the open-pore conductance before and after the event. ( d ) Scatter diagram of the amplitude of the conductance blockade versus translocation time for DNA translocation through a 10-nm diameter nanopore in a graphene monolayer. The accompanying histograms are included at the top and the right. Each point in this scatter diagram corresponds to a single translocation event. Applied voltage is −200 mV. Full size image Characterization of the DNA-antifouling properties In order to estimate the added thickness of the self-assembled monolayer on the graphene, we probed the change in the pore conductance on applying the coating for three pores with diameters of 5, 10 and 15 nm ( Fig. 3e ). Fitting the data according to the model described in Equation 1 would suggest that L increased from 1.5 nm to an apparent thickness L * of 5.5 nm upon forming the self-assembled monolayer. However, the ethylene glycol chains will also protrude into the nanopore area, and therefore the pore will effectively have a smaller diameter d * . If x is the characteristic spatial extent of the pyrene ethylene glycol chains, we obtain a new expression for G(d) by substituting d * =d−2x and L * =L+2x into Equation 1, leading to To estimate the coating thickness x , equation 2 was fitted to the conductance data for the three pores ( d =5, 10 and 15 nm; blue line, Fig. 3e ), adopting the value L =1.5 nm that was obtained before applying the self-assembled monolayer (red line, Fig. 3e ). The result yields a coating thickness x of 0.7±0.2 nm. A value of ~0.7 nm is in good agreement with the estimated sum of the pyrene–graphene spacing (about 0.3 nm) and the persistence length of ethylene glycol molecules in water (about 0.4 nm) (ref. 19 ). The three coated pores reported above were used for translocation experiments with single-stranded DNA. Figure 4 shows the result for the nanopore with a diameter of 10 nm. Single-stranded DNA can be driven electrophoretically through the nanopore and can be detected by monitoring the ion current. Upon addition of the 7-kb long circular M13 single-stranded DNA molecule on one side of the pore and applying a voltage of −200 mV across the graphene membrane, a series of spikes is observed in the conductance traces ( Fig. 4a ). Each temporary drop in the measured conductance, ΔG, arises from a single DNA molecule that translocates through the pore. Two characteristic signals are observed, corresponding to two types of translocation events: type 1 events (where the circular molecule translocates in an non-folded conformation) and type 21 events (where the circular DNA molecule is in a folded conformation), similar to previous reports of DNA translocating through silicon-based nanopores [24] . We focused our study to type 1 event, as those are the most abundant in our data set. Furthermore, they are the most straightforward to interpret because 21 events intrinsically feature a spread in conductance blockade and dwell time. Examples of events are shown in Fig. 4b . From a large number ( n =545) of such events, we obtain a histogram of conductance blockade levels Δ G , as presented in Fig. 4b . Three peaks are visible, the first being the open-pore current at 0 nS (that is, the baseline); the peak at 3.8±0.5 nS that corresponds to one circular M13 molecule in the pore (that is, two parallel single strands); and the peak at 7.5±0.6 nS because of two parts of the same DNA molecule in the pore (that is, four single stands). A scatter plot of Δ G versus the time duration of the events is shown in Fig. 4c . Each dot in this diagram represents a single M13 DNA translocation event. In addition to the event amplitude, we studied the translocation times of the events. The average translocation time is found to be 180±30 μs. These short translocation times are similar to previous reports [6] , [7] , [8] . The same analysis was carried out for the two other nanopores (diameter 5 and 15 nm), and conductance and dwell time histograms are shown in Fig. 5a,b , respectively. Moreover, type 1 translocations are most represented with conductance blockade amplitudes of Δ G 5nm =5.8±0.5 nS and Δ G 15nm =3.4±0.5 nS. The most probable translocation times in the distribution of the events are 250±50 and 135±20 μs for the 5- and 15-nm pore, respectively. Conductance blockades are much larger in amplitude than what is typically observed with silicon nitride nanopore, as expected the thinner graphene membrane [18] . As shown in Fig. 5c , both the conductance blockade and dwell times increase when the diameter of the pores decreases, a trend that was also found for silicon-nitride pores [18] . A fit of Δ G (d) from a model (described in Varghese et al . [20] ) captures the trend in Δ G ( d ) reasonably well, although the graphene nanopores appear to show a somewhat less pronounced dependence of Δ G ( d ) compared with SiN nanopores [20] . 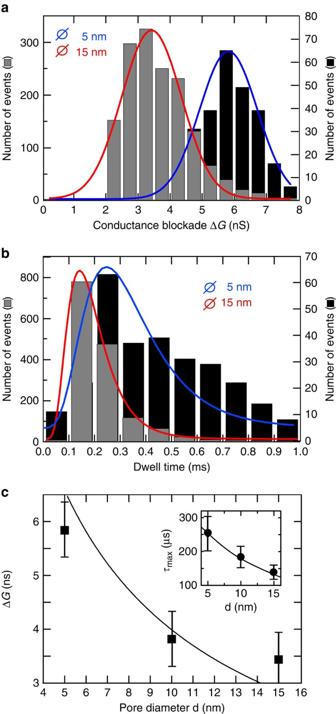Figure 5: DNA translocation through coated 5, 10 and 15 nm graphene nanopores. (a) Conductance blockade histograms from analysing the scatter diagrams for a 5-nm (grey) and 15 nm (black) graphene nanopore. (b) Dwell-time histograms. (c) Conductance blockades and dwell times (inset) versus pore diameter. Black solid line in the main panel represents the best fit of the model of Kowalczyket al.18for ΔG(d) atdssDNA=2.2±0.3 nm, wheredssDNAis the effective diameter of a cylinder that represents the two parallel ssDNA strands of the circular ssDNA. Solid line in the inset is a guide to the eye (error bars derivate from the Gaussian distribution). Figure 5: DNA translocation through coated 5, 10 and 15 nm graphene nanopores. ( a ) Conductance blockade histograms from analysing the scatter diagrams for a 5-nm (grey) and 15 nm (black) graphene nanopore. ( b ) Dwell-time histograms. ( c ) Conductance blockades and dwell times (inset) versus pore diameter. Black solid line in the main panel represents the best fit of the model of Kowalczyk et al . [18] for Δ G ( d ) at d ssDNA =2.2±0.3 nm, where d ssDNA is the effective diameter of a cylinder that represents the two parallel ssDNA strands of the circular ssDNA. Solid line in the inset is a guide to the eye (error bars derivate from the Gaussian distribution). Full size image Our experiments thus show that graphene nanopores can be used to reproducibly detect single DNA molecules without sticking and pore-clogging if the hydrophobicity of graphene is tailored with hydrophilic short ethylene glycol chains. Pores can be measured reproducibly and stably and do not get clogged upon adsorption of double-stranded and single-stranded DNA, although the graphene remains unaltered chemically, which is a prerequisite to the design of future hydrophilic graphene nanopore, nanoribbon and nanogap devices. More generally, we expect that our general approach to tailor graphene into a hydrophilic surface will find its way to a wide range of applications, in which one intends to use graphene in an aqueous environment. How to cite this article: Schneider, G. F. et al . Tailoring the hydrophobicity of graphene for its use as nanopores for DNA translocation. Nat. Commun. 4:2619 doi: 10.1038/ncomms3619 (2013).